Pyrimidine-2,4,6-triones are a new class of voltage-gated L-type Ca2+channel activators Cav1.2 and Cav1.3 are the main L-type Ca 2+ channel subtypes in the brain. Cav1.3 channels have recently been implicated in the pathogenesis of Parkinson’s disease. Therefore, Cav1.3-selective blockers are developed as promising neuroprotective drugs. We studied the pharmacological properties of a pyrimidine-2,4,6-trione derivative (1-(3-chlorophenethyl)-3-cyclopentylpyrimidine-2,4,6-(1H,3H,5H)-trione, Cp8) recently reported as the first highly selective Cav1.3 blocker. Here we show, in contrast to this previous study, that Cp8 reproducibly increases inward Ca 2+ currents of Cav1.3 and Cav1.2 channels expressed in tsA-201 cells by slowing activation, inactivation and enhancement of tail currents. Similar effects are also observed for native Cav1.3 and Cav1.2 channels in mouse chromaffin cells, while non-L-type currents are unaffected. Evidence for a weak and non-selective inhibition of Cav1.3 and Cav1.2 currents is only observed in a minority of cells using Ba 2+ as charge carrier. Therefore, our data identify pyrimidine-2,4,6-triones as Ca 2+ channel activators. L-type Ca 2+ channels (LTCCs, Cav1) represent one of the three major classes (Cav1–3) of voltage-gated Ca 2+ channels [1] . They are expressed in most electrically excitable cells [1] , [2] , [3] . Many physiological processes, including muscle, brain, endocrine and sensory function, depend on proper LTCC activity [2] . Mutant mice and inherited human diseases have provided detailed insight into the physiological and pathophysiological role of these channels [2] , [4] . LTCCs contain high-affinity drug binding sites for dihydropyridines and other chemical classes of organic Ca 2+ channel blockers [5] . Within the L-type Ca 2+ channel family (Cav1.1−Cav1.4), Cav1.2 and Cav1.3 are the main isoforms found in the brain. They are predominantly located at postsynaptic somatodendritic locations, are often present in the same neuron [6] and shape short- and long-term adaptations of synaptic function [2] , [4] , [6] , [7] . However, they are functionally distinct and contribute differently to various brain functions, such as emotional and drug-taking behaviours and different types of memory [2] , [3] , [4] . Cav1.3 comprises only~10% of LTCCs in the brain [8] , but due to its more negative activation voltage range it carries inward current at threshold voltages [9] , [10] . Thereby, it can stabilize upstate potentials, shape firing patterns and contribute to pacemaker currents [2] , [6] , [7] , [11] . L-type Ca 2+ currents also contribute to the dendritic Ca 2+ transients during the autonomous pacemaking in substantia nigra pars compacta (SNc) dopaminergic neurons [12] . These Ca 2+ oscillations add to the increased level of mitochondrial oxidative stress responsible for the particular vulnerability of these neurons to neurodegeneration in Parkinson’s disease (PD) [13] . LTCC blockers can protect these neurons from neurodegeneration in various mammalian PD models [3] , [14] , and epidemiological clinical studies associate the use of brain-permeable Ca 2+ channel blockers in hypertensive patients with reduced PD risk [15] , [16] . Therefore, the inhibition of LTCCs in SNc neurons represents an attractive neuroprotective concept in PD [17] . Currently available LTCC drugs inhibit both Cav1.3 and Cav1.2 (refs 18 , 19 ). Their potent block of Cav1.2 channels in arterial resistance vessels and cardiomyocytes explains their cardiovascular therapeutic benefits but limits their use for neuroprotection in PD [8] . As Cav1.3 channels are also expressed in SNc neurons [20] , there is considerable interest to develop Cav1.3-selective inhibitors as agents for neuroprotection lacking major cardiovascular side effects [17] . A recent study has reported the discovery of pyrimidine-2,4,6-trione derivatives as highly Cav1.3-selective antagonists [17] , [21] . These compounds may not only comprise lead structures for further drug development but also valuable pharmacological tools to dissect the function of Cav1.2 and Cav1.3 for different cellular functions in vivo and in vitro . We have therefore further characterized the pharmacological properties of these compounds and found an unexpected gating modifying effect of Ca 2+ inward currents ( I Ca ) through recombinant and native Cav1.3, as well as Cav1.2 LTCCs. This was characterized by slowing of activation and inactivation kinetics, slowing of deactivation and late inward current stimulation. These pharmacological properties strongly resemble those of the benzoylpyrrole LTCC channel activator FPL64176. Our experiments identify pyrimidine-2,4,6-trione derivatives as a new class of LTCC-activating drugs. Modulation of LTCC Ca 2+ currents by Cp8 The pyrimidine-2,4,6-trione derivatives compound 3 (Cp3; 1-(3-chlorophenethyl)-3-cyclohexylpyrimidine-2,4,6-(1H,3H,5H)-trione) and compound 8 (Cp8; 1-(3-chlorophenethyl)-3-cyclopentylpyrimidine-2,4,6-(1H,3H,5H)-trione) have recently been reported to block rat Cav1.3 channels with low micromolar IC 50 values and with 28– (Cp3) to >100–1,000-fold (Cp8) selectivity over Cav1.2 in fluorometric imaging plate reader and whole-cell patch-clamp assays after stable heterologous expression in HEK-293 cells [17] , [21] . As the permeant ion critically affects LTCC channel kinetics and therefore may affect drug potency and selectivity, we tested these compounds using Ca 2+ as the physiological charge carrier. I Ca inactivates much faster than I Ba by inducing strong Ca 2+ -dependent inactivation (CDI) [22] . Similar to that in the original publication, rat Cav1.3 α1 (rCav1.3 L ) and rabbit Cav1.2 (rbCav1.2 S ) channel constructs were expressed together with β3 and α2δ1 subunits in tsA-201 cells. Cp8 (50 μM) induced a pronounced time-dependent change in current kinetics of both rCav1.3 L and rbCav1.2 S during 0.2 Hz depolarizing pulses from a holding potential (HP) of −80 mV to V max ( Fig. 1a,b ). It was characterized by a slowing of the activation and inactivation time course, accompanied by an increase of tail current. This was due to an increase of peak tail current and a pronounced slowing of deactivation ( Fig. 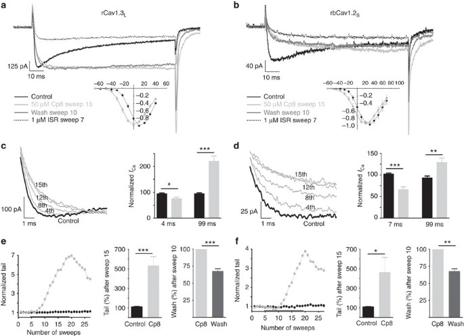Figure 1: Modulation of rCav1.3Land rbCav1.2SCa2+currents by Cp8. ICa(15 mM, 100-ms test pulses toVmaxat 0.2 Hz, HP of −80 mV) through rCav1.3L(a) or rbCav1.2S(b) before, during and after superfusion of the cell with Cp8-containing (50 μM) bath solution. Last sweep before drug application (control) is shown in black. Insets:ICa–Vrelationship before (black) and after (grey) drug application (500-ms long depolarizations to indicated potentials; for statistics seeSupplementary Table 1). Dotted line: ihibition by 1 μM ISR after 7 sweeps. (c,d) Left:ICaduring the first 10 ms of control (left, bold black), 4th, 8th, 12th and 15th (grey) sweep of drug application. Right: effect of 50 μM Cp8 onICathrough rCav1.3L(c,n=14) and rbCav1.2S(d,n=11) at an early (4 ms for rCav1.3L, 7 ms for rbCav1.2S) and late (99 ms) time point. Normalized tail area (per cent of the area under the tail in the presence of drug versus the tail area during the previous control sweeps) of a representative rCav1.3L(e) or rbCav1.2S(f) recording are plotted against the number of sweeps. Left: drug application is indicated by a black line. Middle: normalized tail area (%) after 15 sweeps of drug application for rCav1.3L(e,n=13, range 136–1,259) and rbCav1.2S(f,n=11, range 149–1,874). Right: decrease of tail area (in %) after ten sweeps of subsequent washout with bath solution (rCav1.3L,n=13; rbCav1.2S,n=9). Means±s.e. are shown. Statistical significance was determined using unpairedt-test. ***P<0.001; **P<0.01; *P<0.05. 1a,b ; Table 1 for statistics). The drug also induced an ~10 mV shift in the half-maximal activation voltage ( V 0.5, act ) to more negative voltages (inset Fig. 1a,b ; Supplementary Table 1 ). A steady-state drug effect was usually obtained after 15 pulses (70 s after drug application). This was slower than for inhibition by the dihydropyridine isradipine (ISR; 1 μM), which fully developed profound inhibition within three to nine sweeps ( Fig. 1a,b ). As Cp8 effects were unexpected and previously not reported, we confirmed these findings using three independent supplies of Cp8 (see Methods). We could also rule out drug perfusion artefacts by performing appropriate control experiments (see Methods for detail). Figure 1: Modulation of rCav1.3 L and rbCav1.2 S Ca 2+ currents by Cp8. I Ca (15 mM, 100-ms test pulses to V max at 0.2 Hz, HP of −80 mV) through rCav1.3 L ( a ) or rbCav1.2 S ( b ) before, during and after superfusion of the cell with Cp8-containing (50 μM) bath solution. Last sweep before drug application (control) is shown in black. Insets: I Ca – V relationship before (black) and after (grey) drug application (500-ms long depolarizations to indicated potentials; for statistics see Supplementary Table 1 ). Dotted line: ihibition by 1 μM ISR after 7 sweeps. ( c , d ) Left: I Ca during the first 10 ms of control (left, bold black), 4th, 8th, 12th and 15th (grey) sweep of drug application. Right: effect of 50 μM Cp8 on I Ca through rCav1.3 L ( c , n =14) and rbCav1.2 S ( d , n =11) at an early (4 ms for rCav1.3 L , 7 ms for rbCav1.2 S ) and late (99 ms) time point. Normalized tail area (per cent of the area under the tail in the presence of drug versus the tail area during the previous control sweeps) of a representative rCav1.3 L ( e ) or rbCav1.2 S ( f ) recording are plotted against the number of sweeps. Left: drug application is indicated by a black line. Middle: normalized tail area (%) after 15 sweeps of drug application for rCav1.3 L ( e , n =13, range 136–1,259) and rbCav1.2 S ( f , n =11, range 149–1,874). Right: decrease of tail area (in %) after ten sweeps of subsequent washout with bath solution (rCav1.3 L , n =13; rbCav1.2 S , n =9). Means±s.e. are shown. Statistical significance was determined using unpaired t -test. *** P <0.001; ** P <0.01; * P <0.05. Full size image Table 1 I Ca modulation of different LTCC constructs by Cp8 (50 μ M). Full size table We quantified the drug effect on I Ca at early (at the peak current amplitude in the absence of drug) and late time points (end of test pulse) during the pulse to account for drug-induced changes on current kinetics. Slowing of activation reduced I Ca of rCav1.3 L (quantified after 4 ms depolarization) and of rbCav1.2 S (quantified after 7 ms; Fig. 1c,d ; right panels; Table 1 ). I Ca through both channels was significantly larger at the end of the depolarizing 100-ms pulse, reflecting slowed inactivation ( Fig. 1c,d ; Table 1 ). Fig. 1e,f illustrates the pronounced time-dependent increase of the integrated tail current of a representative cell and the corresponding statistics. Similar data were obtained for human Cav1.3 (hCav1.3 L ) and the carboxy-terminally long rbCav1.2 L (for statistics see Table 1 ). The drug effect was slowly reversible as evident from the constant decrease of integrated tail current ( Fig. 1a,b and e,f , wash) on washout. Inhibition of early inward current was more pronounced for rbCav1.2 S than for rCav1.3 L , but tail currents were similarly increased ( Fig. 1e,f ). The slowing of activation and inactivation, and the increase in late I Ca was also reproducibly ( n =6) illustrated for hCav1.3 L during 5-s depolarizations for control and drug-treated cells ( Fig. 2a ). Slowing of activation kinetics increased the time to peak I Ca and this was again slowly reversible on washout ( Fig. 2b–d ). Taken together, the pharmacological effects of Cp8 on I Ca closely resemble those previously described for the LTCC-activating drug FPL64176 (refs 23 , 24 ) rather than a Ca 2+ channel blocker. Although variable in extent, this modulation was clearly observed in all recordings using Ca 2+ as the charge carrier (>30 cells with Cav1.3 constructs from 6 independent transfections, 16 cells with Cav1.2 constructs from 6 transfections). 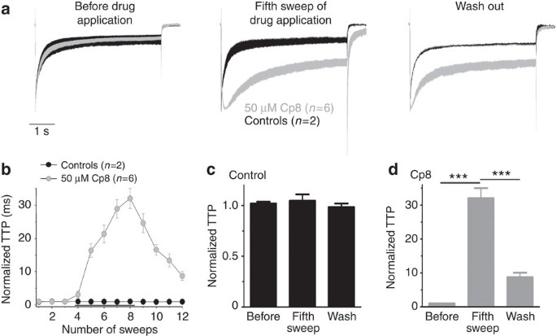Figure 2: Modulation of hCav1.3LICaby Cp8 during 5-s test pulses. (a)ICarecordings of six experiments (5-s depolarizations toVmax, HP −80 mV) were normalized and pooled. Vertical lines represent error bars (means±s.e.).ICabefore, during (5th sweep) and after (4th sweep of washout) superfusion with 50 μM Cp8 is shown. Control cells (black) were perfused with bath solution containing 0.5% (v/v) DMSO. (b) Normalized time to peak (TTP) was plotted against the number of sweeps during drug application (black line) and subsequent washout. Normalized TTP before, during and after superfusion with 50 μM Cp8 (d) or bath solution containing 0.5% (v/v) DMSO (c). Statistical significance was determined using pairedt-test. ***P<0.001. Figure 2: Modulation of hCav1.3 L I Ca by Cp8 during 5-s test pulses. ( a ) I Ca recordings of six experiments (5-s depolarizations to V max , HP −80 mV) were normalized and pooled. Vertical lines represent error bars (means±s.e.). I Ca before, during (5th sweep) and after (4th sweep of washout) superfusion with 50 μM Cp8 is shown. Control cells (black) were perfused with bath solution containing 0.5% (v/v) DMSO. ( b ) Normalized time to peak (TTP) was plotted against the number of sweeps during drug application (black line) and subsequent washout. Normalized TTP before, during and after superfusion with 50 μM Cp8 ( d ) or bath solution containing 0.5% (v/v) DMSO ( c ). Statistical significance was determined using paired t -test. *** P <0.001. Full size image Modulation of LTCC Ba 2+ currents by Cp8 As Ca 2+ channel-activating properties of Cp8 have previously not been observed for the modulation of Ba 2+ currents, we tested whether these kinetic changes were dependent on the permeant ion by repeating the experiments using Ba 2+ as the charge carrier. In 26 of 44 cells expressing rCav1.3 L and 25 of 36 cells (>6 independent transfections) expressing rbCav1.2 S , a very similar kinetic change with a consistent and reversible (on washout) tail current increase was observed as described above for I Ca (cell population labelled ‘Δtail’ in Fig. 3 and Supplementary Table 2 ). Effects on inactivation were less pronounced than for I Ca partly due to the slow voltage-dependent inactivation of I Ba (absence of CDI) ( Fig. 1a,b versus Fig. 3a,b ). Exemplar current traces ( Fig. 3a,b ) as well as statistics for modulation of early and late I Ba and tail current ( Fig. 3e,f ) show again similar modulation of both Cav1.3 and Cav1.2 channels. Comparable effects on tail current were also observed for Cp3 ( Fig. 3e,f , left panels). In addition to the 0.2-Hz pulse protocol, we also applied a protocol (0.05 Hz, 100-ms depolarizations from an HP of −70 mV, external bath solution 2: 10 mM Ba 2+ , see Methods) reproducing the experimental conditions in the original report [17] . The modulatory drug effects were similar using this protocol (for statistics see Supplementary Table 2 ). 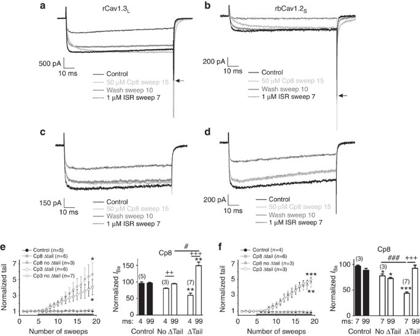Figure 3: Modulation of rCav1.3Land rbCav1.2SBa2+currents by Cp3 and Cp8. Representative traces for modulation of rCav1.3L(a) and rbCav1.2S(b)IBain which tail currents were increased (Δtail) by 50 μM Cp8 (100 ms depolarizations, HP −80 mV toVmax, 0.2 Hz). Last sweep before drug application (control) is shown in black, drug effect is shown 15 sweeps after application and 10 sweeps after starting washout. Dotted line: inhibition by 1 μM ISR after seven sweeps. Arrows indicate the peak of the tail current before drug application. Representative traces of modulation by 50 μM Cp8 of rCav1.3L(c) and rbCav1.2S(d)IBain cells in which no pronounced increase in tail current (no Δtail) was observed. These recordings were analysed separately as described in the text (see alsoTable 2). Same protocol as inaandb,eandf, left: time course of the increase of the tail area for Δtail and no Δtail data sets of rCav1.3L(e) or rbCav1.2S(f). Recordings are shown for Cp8 (grey) and Cp3 (open). Controls were obtained in cells perfused only with bath solution containing 0.5% (v/v) DMSO using the same protocol. Right: effect of 50 μM Cp8 onIBathrough rCav1.3L(e) and rbCav1.2S(f) at an early (4 ms for rCav1.3L, 7 ms for rbCav1.2S) and late (99 ms) time point. Alln-values are given in parentheses. Means±s.e. are shown. Statistical significance was determined using unpairedt-test (control versus Cp8: ***P<0.001; **P<0.01; *P<0.05; Δtail versus no Δtail: ###P<0.001; #P<0.05) or pairedt-test (early versus late time point: +++P<0.001; ++P<0.01). Figure 3: Modulation of rCav1.3 L and rbCav1.2 S Ba 2+ currents by Cp3 and Cp8. Representative traces for modulation of rCav1.3 L ( a ) and rbCav1.2 S ( b ) I Ba in which tail currents were increased (Δtail) by 50 μM Cp8 (100 ms depolarizations, HP −80 mV to V max , 0.2 Hz). Last sweep before drug application (control) is shown in black, drug effect is shown 15 sweeps after application and 10 sweeps after starting washout. Dotted line: inhibition by 1 μM ISR after seven sweeps. Arrows indicate the peak of the tail current before drug application. Representative traces of modulation by 50 μM Cp8 of rCav1.3 L ( c ) and rbCav1.2 S ( d ) I Ba in cells in which no pronounced increase in tail current (no Δtail) was observed. These recordings were analysed separately as described in the text (see also Table 2 ). Same protocol as in a and b , e and f , left: time course of the increase of the tail area for Δtail and no Δtail data sets of rCav1.3 L ( e ) or rbCav1.2 S ( f ). Recordings are shown for Cp8 (grey) and Cp3 (open). Controls were obtained in cells perfused only with bath solution containing 0.5% (v/v) DMSO using the same protocol. Right: effect of 50 μM Cp8 on I Ba through rCav1.3 L ( e ) and rbCav1.2 S ( f ) at an early (4 ms for rCav1.3 L , 7 ms for rbCav1.2 S ) and late (99 ms) time point. All n -values are given in parentheses. Means±s.e. are shown. Statistical significance was determined using unpaired t -test (control versus Cp8: *** P <0.001; ** P <0.01; * P <0.05; Δtail versus no Δtail: ### P <0.001; # P <0.05) or paired t -test (early versus late time point: +++ P <0.001; ++ P <0.01). Full size image In the minority of the cells (18 of 44 cells expressing rCav1.3 L and 11 of 36 cells expressing rbCav1.2 S ), Cp8 and Cp3 inhibited peak I Ba with no consistent and reversible change of tail currents (‘no Δtail’, Fig. 3c,d ). This behaviour was also observed when using the 0.05 Hz protocol ( Supplementary Table 2 ). As this was more compatible with classical Ca 2+ channel block, we analysed these recordings separately to test whether inhibition was Cav1.3 selective. The inhibition of peak I Ba by Cp3 and Cp8 (50 μM) was weak and very similar for both channel isoforms ( Table 2 ), suggesting a lack of Cav1.3 selectivity for Ca 2+ channel-blocking effects under our experimental conditions. Again, the absence or presence of a kinetic change was observed for Cp3 and Cp8 obtained from drug batches synthesized in different laboratories (see Methods). Table 2 I Ba inhibition through rCav1.3 L and rbCav1.2 S by Cp8 (10 and 50 μM) and Cp3 (50 μM) in cells with no consistent and reversible increase in tail current (‘no Δtail’). Full size table Effect of Cp8 on I Ca during fast and brief depolarizations The standard stimulation protocols used so far are suitable to predict the pharmacological modulation of I Ca during long and infrequent depolarizations such as action potentials (APs) in human cardiac myocytes. Therefore, we also quantified the effect of Cp8 on I Ca during shorter (3 ms) stimuli and at high frequency, more closely mimicking electrical activity in the brain ( Fig. 4 ). In contrast to long square pulses, most of the inward current during brief stimuli occurs as tail current on repolarization ( Fig. 4a ). Switching from a stimulation rate of 1 Hz to 100 Hz trains resulted in a reversible decrease of peak tail current through hCav1.3 L during the first 20 sweeps before a new equilibrium was achieved. In control cells, exposure to vehicle only caused a reduction of I Ca without change in current kinetics ( Fig. 4b , left) as expected for I Ca run down. In contrast, Cp8 slowed current activation and tail current decay during individual pulses ( Fig. 4b , right). Peak tail currents during the first pulse were inhibited by the drug ( Fig. 4a,c ) but failed to decrease, and even increased during subsequent pulses, thereby stabilizing larger peak tail currents later during the train ( Fig. 4c ). These experiments confirm the complex modulation of Cav1.3 I Ca during fast trains of depolarization with no evidence for typical LTCC-blocking effects. 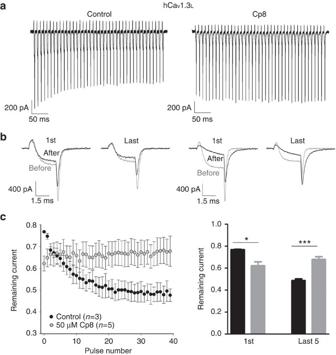Figure 4: Effect of 50 μM Cp8 on hCav1.3LCa2+currents using AP-like stimuli. (a) Representative traces ofICa(15 mM) during 3-ms long depolarizations from an HP of −80 mV to+40 mV with a frequency of 100 Hz after 3 min of drug application (50 μM Cp8, right panel) or perfusion with bath solution containing 0.5% (v/v) DMSO (control, left panel). (b) Current traces illustratingICaduring the first and the last (40th) pulse of AP-like trains before (grey) and after (black) application of drug or control (0.5% (v/v) DMSO) solution in a separate cell. For comparison, traces were normalized to the peak amplitude of the first pulse of one AP-like train before drug application started. (c) Left: mean (±s.e.) change of tail amplitudes during the train in cells treated with control (black) solution or 50 μM Cp8 (grey). Data were normalized to the first action potential before drug application. Right: statistics of remaining current during the first pulse (first) or the mean of the last five pulses (last five) of the trains recorded 3 min after control (black) or Cp8 application (grey). Statistical significance was determined using unpairedt-test. ***P<0.001; *P<0.05. Figure 4: Effect of 50 μM Cp8 on hCav1.3 L Ca 2+ currents using AP-like stimuli. ( a ) Representative traces of I Ca (15 mM) during 3-ms long depolarizations from an HP of −80 mV to+40 mV with a frequency of 100 Hz after 3 min of drug application (50 μM Cp8, right panel) or perfusion with bath solution containing 0.5% (v/v) DMSO (control, left panel). ( b ) Current traces illustrating I Ca during the first and the last (40th) pulse of AP-like trains before (grey) and after (black) application of drug or control (0.5% (v/v) DMSO) solution in a separate cell. For comparison, traces were normalized to the peak amplitude of the first pulse of one AP-like train before drug application started. ( c ) Left: mean (±s.e.) change of tail amplitudes during the train in cells treated with control (black) solution or 50 μM Cp8 (grey). Data were normalized to the first action potential before drug application. Right: statistics of remaining current during the first pulse (first) or the mean of the last five pulses (last five) of the trains recorded 3 min after control (black) or Cp8 application (grey). Statistical significance was determined using unpaired t -test. *** P <0.001; * P <0.05. Full size image Modulation of native LTCCs in mouse chromaffin cells To demonstrate that the channel-activating effects are not only a property of recombinant channel complexes, we also confirmed our findings in mouse chromaffin cells (MCCs) in which we could previously distinguish Cav1.3 and Cav1.2 LTCC components (2 mM Ca 2+ as charge carrier, Fig. 5 ). Under these conditions, 3 μM nifedipine completely block Cav1.2 and Cav1.3, and on average ~50% of the total current is equally carried by Cav1.3 and Cav1.2 in wild-type (WT) mice [10] , [25] . The remaining component is carried by P/Q, N and R-type channels [10] , [26] . Cp8 caused a slight slowing of inactivation during the test pulse ( Fig. 5a , left; b, WT traces) but, as in tsA-201 cells its main effect was a marked prolongation of the tail current. Nifedipine (3 μM) fully blocked this effect ( Fig. 5a ). Tails at −50 mV in the presence of nifedipine and nifedipine+Cp8 were indistinguishable ( n =7), suggesting that the modulation is limited to LTCCs. Deactivation of control currents occurred mono-exponentially with a single, submillisecond time constant ( τ fast ), while in the presence of Cp8 it followed a double-exponential time course with a fast ( τ fast ) and a slow component ( τ slow ) ( Fig. 5b , right, repolarization to −40 mV). τ slow was an order of magnitude slower and contributed maximally to deactivation during repolarization voltages ( V r ) of −50 or −40 mV ( Fig. 5b , n =7). τ fast was not affected by Cp8 ( Fig. 5b ). To determine whether Cav1.2 channels are modulated by the drug, we repeated these experiments in Cav1.3-deficient mice (Cav1.3 −/− , n =6) that only express Cav1.2 LTCCs. Slowing of tail currents was also evident in Cav1.3 −/− cells ( Fig. 5b ). Again, τ slow was about an order of magnitude slower than τ fast but significantly smaller (2.6 versus 3.3 ms) than in WT, indicating a slightly less-pronounced potentiating action of Cp8 on Cav1.2 channels. The slow kinetic component also contributed less to the total tail current amplitude in Cav1.3 −/− MCCs (15.5% (red triangles) versus 25.5% (red circles) in Fig. 5b middle). This lower contribution is compatible with the absence of Cp8-modified Cav1.3 channels in Cav1.3 −/− mice. 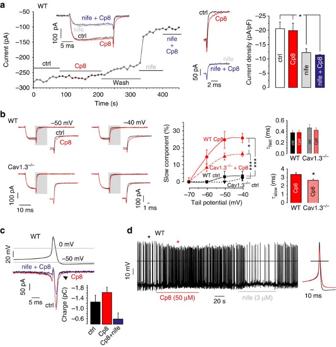Figure 5: Modulation of LTCC currents in MCCs. (a) Left: time course of peakICaamplitude of a representative MCC (HP −50 mV, test potential 0 mV) before, during and after perfusion with control or drug-containing solutions (nifedipine 3 μM, Cp8 50 μM) as indicated. Inset: current traces before and during steady-state drug effects. Middle: tail currents at −50 mV on an expanded time scale. Right:ICadensity at the test pulse (0 mV) (n=7). (b) Left: examples of current traces (0 mV) with repolarization (Vr) to either −50 or −40 mV in WT and Cav1.3−/−MCCs. Middle: control tails were fast and mono-exponential while Cp8 tails showed double-exponential decay with a fast (τfast) and a slow component (τslow) with voltage-dependent contribution. The percentage of the slow component amplitude versusVris illustrated for WT (n=7) and Cav1.3−/−MCCs (n=6). In the absence of Cp8, the slow component is absent in most cells. Right:τfastat −40 mV was not affected by Cp8 in both WT and Cav1.3−/−MCCs.τslowwas only evident in the presence of Cp8. (c) Effects of Cp8 onICaduring an AP clamp. The potentiating effect of Cp8 is more evident on the repolarizing phase (post-AP tails) than during the pacemaking (pre-AP). The changes of total Ca2+charge are given in the inset. (d) Cp8 increases spontaneous firing frequency (from 0.7±0.2 Hz (control) to 1.3±0.2 Hz (Cp8),n=6,P<0.05, pairedt-test), in contrast to nifedipine (3 μM), which reduces or blocks the firing. Right: single action potential before and during Cp8 perfusion. One of six representative experiments is shown. The afterhyperpolarization decreases from −47.8±2.4 mV (control) to −42.9±−2.7 (Cp8) (P<0.05), and the overshoot decreases from 14.4±4.1 mV (control) to 6.5±4.5 mV (Cp8) (n=6,P<0.001, pairedt-test). Cp8 also causes a widening of the AP half width from 4.7±0.6 ms to 9.8±2.2 ms (P<0.05). Figure 5: Modulation of LTCC currents in MCCs. ( a ) Left: time course of peak I Ca amplitude of a representative MCC (HP −50 mV, test potential 0 mV) before, during and after perfusion with control or drug-containing solutions (nifedipine 3 μM, Cp8 50 μM) as indicated. Inset: current traces before and during steady-state drug effects. Middle: tail currents at −50 mV on an expanded time scale. Right: I Ca density at the test pulse (0 mV) ( n =7). ( b ) Left: examples of current traces (0 mV) with repolarization ( V r ) to either −50 or −40 mV in WT and Cav1.3 −/− MCCs. Middle: control tails were fast and mono-exponential while Cp8 tails showed double-exponential decay with a fast ( τ fast ) and a slow component ( τ slow ) with voltage-dependent contribution. The percentage of the slow component amplitude versus V r is illustrated for WT ( n =7) and Cav1.3 −/− MCCs ( n =6). In the absence of Cp8, the slow component is absent in most cells. Right: τ fast at −40 mV was not affected by Cp8 in both WT and Cav1.3 −/− MCCs. τ slow was only evident in the presence of Cp8. ( c ) Effects of Cp8 on I Ca during an AP clamp. The potentiating effect of Cp8 is more evident on the repolarizing phase (post-AP tails) than during the pacemaking (pre-AP). The changes of total Ca 2+ charge are given in the inset. ( d ) Cp8 increases spontaneous firing frequency (from 0.7±0.2 Hz (control) to 1.3±0.2 Hz (Cp8), n =6, P <0.05, paired t -test), in contrast to nifedipine (3 μM), which reduces or blocks the firing. Right: single action potential before and during Cp8 perfusion. One of six representative experiments is shown. The afterhyperpolarization decreases from −47.8±2.4 mV (control) to −42.9±−2.7 (Cp8) ( P <0.05), and the overshoot decreases from 14.4±4.1 mV (control) to 6.5±4.5 mV (Cp8) ( n =6, P <0.001, paired t -test). Cp8 also causes a widening of the AP half width from 4.7±0.6 ms to 9.8±2.2 ms ( P <0.05). Full size image The activating properties of Cp8 were also confirmed on Ca 2+ currents during an AP clamp in WT MCCs. The potentiating effect of Cp8 is more evident on the repolarizing phase (post-AP; tails) than during the pacemaking (pre-AP) and caused an increase in total Ca 2+ charge during the AP ( Fig. 5c , n =5). As expected from its channel-activating properties, Cp8 nearly doubled the spontaneous firing frequency of MCCs, in contrast to nifedipine that either decreased or blocked the firing [10] ( n =6, for statistics see Fig. 5d ). This was accompanied by a Cp8-induced reduction of the after-hyperpolarization of the AP ( Fig. 5d , right). The unexpected finding of our study was the absence of any evidence for a Cav1.3-selective Ca 2+ channel-blocking effect of Cp3 and Cp8, two compounds recently claimed to be highly Cav1.3-selective channel blockers in fluorometric imaging plate reader and patch-clamp studies [17] , [27] . Our results also differed from those previously published, because we observed (non-selective) current inhibition only in the minority of experiments and only using Ba 2+ as a charge carrier. Instead, in most experiments with Ba 2+ and in all experiments using Ca 2+ as the charge carrier, Cp8 reproducibly induced pronounced changes of current kinetics through rbCav1.2 S and rCav1.3 L expressed in tsA-201 cells. These changes were characterized by a slowing of the activation and inactivation time course during depolarizing stimuli. They were observed in independent transfections, were independent of current size, could be slowly washed out in most cells and were also observed with experimental conditions (composition of bath solution, stimulation protocol), reproducing those described in the original publication [17] . As described in Methods, we also took special care to rule out experimental artefacts such as drug carryover, pharmacological effects of chemicals eluting from plastic material [28] or dimethyl sulphoxide (DMSO) effects. As we performed control experiments in separate cells using the same stimulation protocol and application time course, we also fully accounted for changes in current kinetics and amplitude (including current run down) not mediated by the test compounds. Moreover, the characteristic kinetic changes were reproducibly observed not only with the compounds synthesized in our laboratory but also from two other independent sources (Methods). The channel constructs used for our study were the same (Cav1.2) or very similar (Cav1.3) to those described in the original report. Their integrity was verified by DNA sequencing and also resulted in the L-type current characteristics expected for the two channel isoforms. Cav1.3 currents activated at more negative voltages than Cav1.2 ( Supplementary Table 3 ) and exhibited an initial faster inactivating component (due to more pronounced CDI [29] ) with Ca 2+ as the charge carrier ( Fig. 1a,b ). As the C terminus of Cav1.2 can also be proteolytically cleaved and can even be released from the channel into the nucleus as independent transcriptional regulator [3] , [30] , [31] , we tested both long and short Cav1.2 α1-subunit variants, without an obvious difference in Cp8 response. We also observed no relevant difference between the rat and human Cav1.3 constructs. Unexpectedly, the modulation of I Ca by Cp8 closely resembled the actions of the LTCC activator FPL64176. This drug also slows activation and inactivation kinetics, increases peak current and slows current deactivation [23] , [24] , [32] , [33] . It is therefore possible that despite its unrelated structure, channel modulation of I Ca by Cp8 occurs through similar mechanisms than by FPL64176. This includes the possibility that Cp8 stabilizes a conducting inactivated state that can explain the slowing of current kinetics [23] . However, one notable difference is that in a minority of cells, and only with Ba 2+ as charge carrier, the effects on tail currents were virtually absent and weak, and non-selective Ca 2+ channel-blocking effects by Cp8 (and Cp3) were evident. Application of 50 μM caused <30% inhibition of I Ba . This is in contrast to a reported IC 50 of ~25 μM in similar patch-clamp experiments [17] . Notably, the extent of inhibition of rbCav1.2 S by Cp8 was comparable with the data previously reported for Cav1.2, suggesting that the absence of selectivity for blocking effects in our experiments resulted from a lower apparent sensitivity of Cav1.3. The absence or presence of a kinetic change was not predicted by current amplitudes and both behaviours (with or without tail current changes) could be observed even within the same transfection and the same day of I Ba recording. Currently, we cannot explain the differences between our data and those reported for both compounds previously [17] . One possibility is that the stable rat Cav1.3 cell line that has been used for the initial characterization displays abnormally high sensitivity towards these compounds. This could result from the selection of a suitable clone from a large number of clones. To our knowledge the biophysical and pharmacological properties of this stable clone have never been reported in detail. This appears to be important because an earlier study using a stable Cav1.3-expressing cell line also could not detect essential biophysical hallmarks of Cav1.3, such as its negative activation voltage range [34] . Here we used transiently transfected cells. Although this may introduce additional variability, it is more suitable to reveal the true spectrum of pharmacological properties of these channels. As we found (weak) Ca 2+ channel-blocking activity by these compounds in a population of cells with Ba 2+ recordings, it is possible that channel blocking by Cp8 depends on a certain channel state that is preferentially stabilized by Ba 2+ and/or favoured in some stable cell lines. The voltage-dependent widening of the L-type I Ca tail component in MCCs proves that the channel-activating properties of Cp8 also apply to native LTCCs. As we found no evidence for I Ca inhibition or tail current slowing by Cp8 in the presence of nifedipine, we provide evidence that Cp8 effects spare non-LTCCs (which comprise about half of the I Ca in MCCs under our experimental conditions [10] , [26] ). In contrast to tsA-201-expressed channels we found no clear effects on I Ca kinetics and whole-cell current amplitudes during our brief test pulses, although a slight slowing of inactivation during depolarization was evident in some cells. However, changes of current kinetics are more difficult to quantify in MCCs because of the large contribution of non-LTCCs to I Ca . In Cav1.3 −/− MCCs where Cav1.2 remains as the only LTCC [10] , [25] , we still observed Cp8-induced appearance of a slowly decaying tail current component demonstrating that the drug also modulates native Cav1.2 channels. In AP-clamp configuration, plenty of Ca 2+ current is conducted during the tail currents on AP repolarization. Cp8 widened this Ca 2+ -tail component in all tested cells ( n =6) and augmented the Ca 2+ current charge. Using Cav1.3 −/− mice, we have previously identified Cav1.3 LTCCs as critical pacemaker channels in MCCs [10] , [25] . The LTCC-activating effect of Cp8 can therefore also explain the drug-induced increase in spontaneous firing frequency of MCCs observed in our experiments. This was accompanied by a reduced after-hyperpolarization of the MCC AP in the presence of drug. We hypothesize that this is due to the specific increase of I Ca during the tails. At this point the large-conductance, Ca 2+ -activated potassium channels (voltage sensitive) are about to close; thus, the effect of the increased tail I Ca will be a reduced net outward current that will contribute to a depolarization [35] . However, we cannot rule out Cp8 effects on K + channels as well. In accordance with our results obtained in tsA-201 cells, we have no evidence for Ca 2+ channel-blocking effects of Cp8 in MCCs. Taken together, we conclude that Cav1.3-selective compounds reproducibly inhibiting LTCCs independent of experimental conditions and devoid of Ca 2+ channel-activating properties still need to be discovered. The large number of pyrimidine-2,4,6-triones that has been generated in previous studies [17] , [21] should comprise a suitable library to screen for lead compounds of Cav1.3-selective blockers. Our finding that Cp8 appears to spare non-LTCCs suggests that such compounds specifically target a binding pocket present only on LTCCs. Electrophysiological recordings in tsA-201 cells tsA-201 cells (a human embryonic kidney cell line stably expressing a SV40 temperature sensitive T antigen, ECACC, 96121229) were cultured in DMEM supplemented with 10% FCS (Gibco, 10270-106), 2 mM L -glutamine (Gibco, 25030-032), penicillin (10 units per ml; Sigma, P-3032) and streptomycin (10 μg ml −1 ; Sigma, S-6501), and maintained at 37 °C in a humidified incubator with 5% CO 2 . Cells were grown and split when they reached ~80% of confluence using 0.05% trypsin for cell dissociation. The cell’s passage number did not exceed 20 passages. For whole-cell patch-clamp recordings, tsA-201 cells were transiently transfected with an equimolar ratio of complementary DNA encoding full-length α1-subunits together with auxiliary β3 (rat, NM_012828) and α2δ1-subunits (rabbit, NM_001082276) [9] , [18] using Ca 2+ -phosphate. Briefly, 0.5 ml of DNA in CaCl 2 (250 mM CaCl 2 ) was added dropwise to 0.5 ml HEBS (274 mM NaCl, 40 mM HEPES, 10 mM KCl, 1.4 mM Na 2 HPO 4 × 2H 2 O, 12 mM dextrose, pH 7.05) at 37 °C. The mix was then incubated at room temperature for 20 min and the precipitates formed were added directly drop by drop to cells. Medium was changed after 6–8 h incubation at 37 °C and 5% CO 2 . To visualize transfected cells, green fluorescent protein was co-transfected. Cells were then plated onto a 35-mm culture dish pre-coated with poly- L -lysine. The cells were kept at 30 °C and 5% CO 2 , and subjected to electrophysiological measurements 48–72 h after transfection. For whole-cell patch-clamp recordings, electrodes with a resistance of 2–5 MΩ were pulled from glass capillaries (Borosilicate glass, 64-0792, Harvard Apparatus, USA) using a micropipette puller (Sutter Instruments) and fire-polished with an MF-830 microforge (Narishige, Japan). Cells were recorded in the whole-cell configuration using Axopatch 200A amplifier (Axon Instruments, Foster City, CA). Recordings were digitized (Digidata 1322A digitizer, Axon Instruments) at 50 kHz, low-pass filtered at 5 or 2 kHz and subsequently analysed using pClamp 10.2 software (Axon Instruments). Experiments showing currents bigger than 3 nA were prospectively excluded from analysis. Linear leak and capacitative currents were subtracted offline (5-s pulses, 100 ms protocol) or online (P/4 protocol). Compensation was applied for 60–70% of the series resistance. The pipette internal solution contained (in mM): 135 CsCl, 10 HEPES, 10 Cs-EGTA, 1 MgCl 2 , 4 ATP-Na 2 adjusted to pH 7.4 with CsOH (311 mOsm l −1 ); bath solution 1 (for 0.2 Hz recordings) contained (in mM): 15 BaCl 2 , 10 HEPES, 150 Choline-Cl and 1 MgCl 2 , adjusted to pH 7.4 with CsOH; bath solution 2 (for 0.05 Hz recordings) contained (in mM): 10 BaCl 2 , 140 NaCl, 1 MgCl 2 , 10 HEPES, 20 CsCl adjusted to pH 7.4 with CsOH, osmolarity ~320 mOsm l −1 ; bath solution 3 contained (in mM): 15 CaCl 2 , 10 HEPES, 150 Choline-Cl, and 1 MgCl 2 , adjusted to pH 7.4 with CsOH; current–voltage ( I – V ) relationships were obtained by applying a 20- or 500-ms long square pulse protocol (as indicated in the figure legends) to various test potentials starting from an HP of −80 mV. Resulting I – V curves were fitted to the equation I = G max ( V − V rev )/{1+exp[−( V − V 0.5,act )/ k act ]} where I is the peak current amplitude, G max is the maximum slope conductance, V is the test potential, V rev is the extrapolated reversal potential, V 0.5,act is the half-maximal activation voltage and k act is the slope factor. Ba 2+ or Ca 2+ currents were recorded using either a 0.2-Hz protocol (100 ms test pulses to V max , HP −80 mV, bath solution 1 and 3) or a 0.05 Hz protocol (100 ms test pulses to V max , HP −70 mV, bath solution 2). For the quantification of tail currents, the area under the curve between the peak of the tail current and the subsequent 17 ms was integrated. Five-second long square pulses were elicited from an HP of −80 mV to V max every 30 s. AP-like square stimuli: 3 ms from an HP of −80 mV to+40 mV with a frequency of 1 or 100 Hz. Drug perfusion Concentrations (50 μM) of drug were routinely employed to ensure fast equilibrium of the slow drug effects and because lower concentrations produced only minimal effects on I Ba ( Table 2 ). Cells were perfused by an air pressure-driven perfusion system (BPS-8 Valve Control System, ALA Scientific Instruments) with external solutions in the presence or absence of drugs with a flow rate of 0.6 ml min −1 . Drug application was started after at least four constant control sweeps during perfusion with external bath solution. To ensure that the perfusion system was not contaminated, each day before measuring the compounds, individual control recordings with only bath solution containing 0.5% (v/v) DMSO were performed, using the tubes subsequently used for test compounds. The recording setup and perfusion system has never been exposed to Ca 2+ channel activators (such as BayK8644 or FPL64176). Complete exchange of the solution around the perfused cell was obtained in <50 ms. All experiments were performed at room temperature (~25 °C). Electrophysiological recordings from MCCs Chromaffin cells were isolated and dissociated from 3-month-old male C57BL/6N or male Cav1.3 −/− mice as described in detail previously [10] , [25] . Ethical approval was obtained for all experimental protocols from the University of Torino Animal Care and Use Committee, Torino, Italy. All experiments were conducted in accordance with the National Guide for the Care and Use of Laboratory Animals adopted by the Italian Ministry of Health. A drop (100 μl) of concentrated cell suspension was plated on poly-ornithine (1 mg ml −1 ; Sigma-Aldrich, Munich, Germany) and laminin (5 μg ml −1 ; Sigma-Aldrich, Munich, Germany) coated petri-dishes and 30 min later 1.9 ml of DMEM containing 1% penicillin/streptomycin (Sigma-Aldrich) and 15% FCS (Sigma-Aldrich) was added. The primary chromaffin cell culture was kept in an incubator at 37 °C and water saturated atmosphere with 5% CO 2 . Currents were recorded in perforated-patch conditions using a multiclamp 700-B amplifier and pClamp 10.0 software (Molecular Devices, Sunnyvale, CA, USA) [10] , [25] . Traces were filtered using a low-pass Bessel filter set at 1–2 kHz and sampled at 10 kHz using a digidata 1440 A acquisition interface (Molecular Devices). Borosillicate glass pipettes (Kimble Chase life science, Vineland, NJ, USA) with a resistance of 2–3 MΩ were dipped in an Eppendorf tube containing intracellular solution before being back-filled with the same solution containing 500 μg/ml of amphotericin B (Sigma-Aldrich) dissolved in DMSO (Sigma-Aldrich). Recordings were initiated after amphotericin B brought the access resistance below 15 MΩ (5–10 min). Series resistance was compensated by 80% and monitored throughout the experiment. Fast capacitive transients during step-wise depolarizations (in voltage clamp) were minimized online by the patch-clamp analogue compensation. Uncompensated capacitive currents (in voltage clamp) were further reduced by the subtraction of the averaged currents in response to P/4 hyperpolarising pulses. Intracellular solution used for Ca 2+ current measurements was (in mM): 135 Cs-MeSO 3 , 8 NaCl, 2 MgCl 2 and 20 HEPES, pH 7.4 (with CsOH). The extracellular solution was (in mM): 135 TEACl, 2 CaCl 2 , 2 MgCl 2 , 10 HEPES, 10 glucose, pH 7.4 (with TEA-OH). TTX (300 nM; Tocris Bioscience: Bristol, UK) was added to avoid contamination by Na + currents. Intracellular solution for current clamp was (in mM): 135 KAsp, 8 NaCl, 20 HEPES, 2 MgCl 2 , 5 EGTA, pH 7.4 (with NaOH; Sigma-Aldrich). The extracellular solution used for current clamp measurements is based on a physiological Tyrode’s solution containing in mM: 30 NaCl, 4 KCl, 2 CaCl 2 , 4 MgCl 2 , 10 HEPES and 10 glucose, pH 7.4 (with NaOH). Nifedipine (nife) was obtained from Sigma Chemicals (N7634). Nifedipine as well as Cp8 were dissolved in DMSO to stock concentrations of 1 and 50 mM, respectively, and used in final concentrations of 3 and 50 μM, respectively. cDNA constructs Full-length rat rCav1.3 L corresponds to GenBank accession number AF370010 / AF370009 (long C terminus) containing exon 31A instead of exon 31, and with the prototypical rat Cav1.3 α1 subunit sequence as predicted from the genomic sequence (7M2K motif at amino terminus, Gly in position 244, Ala in 1,104 and Val in 2,075; for details see ref. 36 ); full-length rabbit rbCav1.2 L : GenBank accession number X15539 (same as P15381 used by Kang et al . [17] ); rbCav1.2 S : rbCav1.2 L truncated at position Δ1800 (refs 30 , 37 , 38 ); human full-length hCav1.3 L : GenBank accession number EU363339 . The short form of Cav1.2 lacks 371 C-terminal amino acid residues, which are believed to be cleaved off by posttranslational proteolytic processing from a portion of the Cav1.2 α1 subunits. This stable fragment can dissociate from the channel and serve as transcriptional regulator or remains bound mediating regulation by protein kinase-A [3] . Our human and rat α1 subunit constructs are highly conserved (>95% sequence identity, most of the difference resulting from the absence of short exons 11 and 44 in human clone) and are functionally indistinguishable [36] . Assuming that non-natural point mutations have been corrected in the clones used for generating stable cell lines used in the original report [39] , our rCav1.3 L construct differs from the rat α1 construct used by Kang et al . [17] only in exon 31 and 9 N-terminal residues, which should cause only minimal functional differences (as reported in ref. 36 ). Solutions and chemicals ISR was obtained from Sigma Chemicals (ISR: I6658). The pyrimidine-2,4,6-trione derivatives Cp3 and Cp8 (labeling according to Kang et al . [17] ) were synthesized as described below. Compounds were independently obtained as a gift from Dr Tuck Soong and from Boehringer Ingelheim Pharma GmbH & Co. KG, Biberach, Germany. Stock solutions (10 mM) of Cp3, Cp8 and ISR were prepared in DMSO (maximum final concentration of 0.5% (v/v)). DMSO did not affect Cav1.3 and Cav1.2 channel currents as shown in control experiments carried out with active drug perfusion protocols (‘controls’ in Figures and Tables). Drugs were diluted to the indicated final concentrations before experiments. Synthesis of Cp3 and Cp8 To a stirred solution of 0.272 g (150 mmol) 1-chloro-3-(2-isocyanatoethyl)benzene in anhydrous methylene chloride (15 ml), 1.50 mmol of the appropriate amine was added. After stirring for 5 h at room temperature, 0.233 g (1.65 mmol) of malonyl dichloride dissolved in 75 ml of anhydrous methylene chloride was added dropwise over 5 min under vigorous stirring. The solution was stirred for another 1 h at room temperature. The solvent was removed under reduced pressure. Purification was performed by column chromatography using 50 g of silica gel and petroleum ether/ethyl acetate (2:8). Cp3: derived from 0.149 g (1.50 mmol) cyclohexanamine. The reaction afforded 0.301 g (0.86 mmol) as a white powder (yield: 58%); m.p. : 154–155 °C; 1 H-NMR (200 MHz, CDCl 3 ): δ 7.28–7.10 (m, 4 H), 4.60 (m, 1H), 4.14–4.00 (m, 2H), 3.61 (s, 2H), 2.95–2.80 (m, 2H), 2.36–2.12 (m, 2H), 1.94–1.76 (m, 2H), 1.74–1.53 (m, 3H), 1.48–1.15 (m, 3H); 13 C-NMR (50 MHz, CDCl 3 ): δ 164.8, 164.7, 151.3, 140.0, 134.5, 130.0, 129.3, 127.3, 127.1, 55.6, 42.8, 40.4, 33.8, 29.2, 26.5, 25.3; high resolution mass spectrometry (electrospray ionization (ESI)) calculated for C 18 H 21 ClN 2 O 3 [M-H] − : 347.1168, found 347.1213. Cp8: derived from 0.128 g (1.50 mmol) cyclopentanamine. The reaction afforded 0.363 g (1.08 mmol) as an off-white powder (yield: 72%); m.p. : 131–132 °C; 1 H-NMR (200 MHz, CDCl 3 ): δ 7.29–7.09 (m, 4H), 5.24–5.02 (m, 1H), 4.15–4.00 (m, 2H), 3.63 (s, 2H), 2.95–2.80 (m, 2H), 2.60–1.72 (m, 6H), 1.71–1.48 (m, 2H); 13 C-NMR (50 MHz, CDCl 3 ): δ 164.9, 164.7, 151.1, 140.0, 134.5, 130.0, 129.3, 127.3, 127.1, 54.5, 42.8, 40.3, 33.9, 28.9, 25.7; high resolution mass spectrometry (ESI) calculated for C 17 H 19 ClN 2 O 3 [M-H] − : 333.1011, found 333.1052. All starting materials were obtained from Sigma-Aldrich. Reactions were monitored by thin-layer chromatography using Polygram SIL G/UV254 (Macherey-Nagel) plastic-backed plates (0.25 mm layer thickness) and visualized using an ultraviolet lamp. Column chromatography was performed using silica gel 60 (0.040–0.063 mm). The identity of both compounds was confirmed by 1 H-NMR, 13 C-NMR and ESI-mass spectrometry (MS). 1 H- and 13 C-NMR spectra were recorded from CDCl 3 solutions on a Varian Gemini 2000 (200 and 50 MHz, respectively) spectrometer using tetramethylsilane as internal standard. Chemical shifts are given in p.p.m. (for details see Supplementary Figs 1 and 2 ). ESI-MS measurements were acquired on a microTOF-Q II mass spectrometer (Bruker-Daltonics, Bremen, Germany). MS parameters: ESI, Nebulizer gas 23.2 psi, dry gas 8.0 l min −1 at 200 °C, capillary voltage 4.5 kV. The mass scan range was set to 100–1,000 m / z with a scan rate of 1 Hz ( Supplementary Figs 3 and 4 ). Purity of both compounds was confirmed via HPLC using a Shimadzu HPLC-System equipped with SIL-20A HT Auto Sampler, CTO-10-AS VP Column Oven, DGU-20A3 Degasser, SPD-M20A Diode Array Detector and two LC-20AD pumps. The column was a 250 × 4-mm Eurospher 100-5 C-18 column with precolumn from Knauer. The mobile phase consisting of acetonitrile/water (3:1) had a constant flow rate of 1 ml min −1 at 24 °C. Compounds were detected at 225 nm. HPLC showed a purity of>98% via integration of area under the peak ( Supplementary Figs 5 and 6 ). Statistics Data analysis was performed using Clampfit 10.2 (Axon Instrumens) and Sigma Plot 11 (Systat Software Inc.). All values are presented as mean±s.e. for the indicated number of experiments ( n ). Data were analysed by unpaired or paired t -test as indicated for individual experiments using Graph Pad Prism 5.1 software (GraphPad Software Inc.). Statistical significance was set at P <0.05. How to cite this article: Ortner, N. J. et al . Pyrimidine -2,4,6-triones are a new class of voltage-gated L-type Ca 2+ channel activators. Nat. Commun. 5:3897 doi: 10.1038/ncomms4897 (2014).